Network physiology reveals relations between network topology and physiological function The human organism is an integrated network where complex physiological systems, each with its own regulatory mechanisms, continuously interact, and where failure of one system can trigger a breakdown of the entire network. Identifying and quantifying dynamical networks of diverse systems with different types of interactions is a challenge. Here we develop a framework to probe interactions among diverse systems, and we identify a physiological network. We find that each physiological state is characterized by a specific network structure, demonstrating a robust interplay between network topology and function. Across physiological states, the network undergoes topological transitions associated with fast reorganization of physiological interactions on time scales of a few minutes, indicating high network flexibility in response to perturbations. The proposed system-wide integrative approach may facilitate the development of a new field, Network Physiology. Physiological systems under neural regulation exhibit high degree of complexity with non-stationary, intermittent, scale-invariant and nonlinear behaviours [1] , [2] . Moreover, physiological dynamics transiently change in time under different physiological states and pathologic conditions [3] , [4] , [5] , in response to changes in the underlying control mechanisms. This complexity is further compounded by various coupling [6] , [7] and feedback interactions [8] , [9] , [10] among different systems, the nature of which is not well-understood. Quantifying these physiological interactions is a challenge as one system may exhibit multiple simultaneous interactions with other systems where the strength of the couplings may vary in time. To identify the network of interactions between integrated physiological systems, and to study the dynamical evolution of this network in relation to different physiological states, it is necessary to develop methods that quantify interactions between diverse systems. Recent studies have identified networks with complex topologies [11] , [12] , [13] , and have focused on emergence of self-organization and complex network behaviour out of simple interactions [14] , [15] , [16] , [17] , network robustness [18] , [19] , [20] , and, more recently, critical transitions due to failure in the coupling of interdependent networks [21] . Growth dynamics of structural networks have been investigated in network models [11] , [13] , and in physical systems [13] , [22] , and various structural and functional brain networks have been explored [22] , [23] . However, understanding the relationship between topology and dynamics of complex networks remains a challenge, especially when networks are comprised of diverse systems with different types of interaction, each network node represents a multicomponent complex system with its own regulatory mechanism, the output of which can vary in time, and when transient output dynamics of individual nodes affect the entire network by reinforcing (or weakening) the links and changing network topology. A prime example of a combination of all these network characteristics is the human organism, where integrated physiological systems form a network of interactions that affects physiological function, and where breakdown in physiological interactions may lead to a cascade of system failures [24] . We investigate the network of interactions between physiological systems, and we focus on the topology and dynamics of this network and their relevance to physiological function. We hypothesize that during a given physiological state, the physiological network may be characterized by a specific topology and coupling strength between systems. Further, we hypothesize that coupling strength and network topology may abruptly change in response to transition from one physiological state to another. Such transitions may also be associated with changes in the connectivity of specific network nodes, that is, the number of systems to which a given physiological system is connected can change, forming subnetworks of physiological interactions. Probing physiological network connectivity and the stability of physiological coupling across physiological states may thus provide new insights on integrated physiological function. Such a system-wide perspective on physiological interactions, tracking multiple components simultaneously, is necessary to understand the relationship between network topology and function. Time delay stability and network of physiological interactions The framework we propose is based on a complex networks approach to quantify physiological interactions between diverse physiological systems, where network nodes represent different physiological systems and network links indicate the dynamical interaction (coupling) between systems. This framework allows to quantify the topology and the associated dynamics in the links strength of physiological networks during a given physiological state, taking into account the signal output of individual physiological systems as well as the interactions among them, and to track the evolution of multiple interconnected systems undergoing transitions from one physiological state to another ( Fig. 1 ). We introduce the concept of time delay stability (TDS) to identify and quantify dynamic links among physiological systems. We study the network of interactions for an ensemble of key integrated physiological systems (cerebral, cardiac, respiratory, ocular and muscle activity). We consider different sleep stages (deep, light, rapid eye movement (REM) sleep and quite wake) as examples of physiological states. While earlier studies have identified how sleep regulation influences aspects of the specific control mechanism of individual physiological systems (for example, cardiac or respiratory [3] , [4] , [25] , [26] ) or have focused on the organization of functional connectivity of electroencephalogram (EEG) networks during sleep [27] and under neurological disorders such as epilepsy [28] , the dynamics and topology of a physiological network comprised of diverse systems have not been studied so far. Further, the relationship between network topology and function, and how it changes with transitions across distinct physiological states is not known. We demonstrate that sleep stages are associated with markedly different networks of physiological interactions ( Fig. 2 ) characterized by different number and strength of links ( Figs 3 and 4 ), by different rank distributions ( Fig. 5 ) and by specific node connectivity ( Fig. 6 ). Traditionally, differences between sleep stages are attributed to modulation in the sympatho-vagal balance with dominant sympathetic tone during wake and REM [25] : spectral, scale-invariant and nonlinear characteristics of the dynamics of individual physiological systems indicate higher degree of temporal correlations and nonlinearity during wake and REM compared with non-REM (light and deep sleep) where physiological dynamics exhibit weaker correlations and loss of nonlinearity [3] , [26] . In contrast, the network of physiological interactions shows a completely different picture: the network characteristics during light sleep are much closer to those during wake and very different from deep sleep ( Figs 2 and 3 ). Specifically, we find that network connectivity and overall strength of physiological interactions are significantly higher during wake and light sleep, intermediate during REM and much lower during deep sleep. Thus, our empirical observations indicate that while sleep-stage-related modulation in sympatho-vagal balance has a key role in regulating individual physiological systems, it does not account for the physiological network topology and dynamics across sleep stages, showing that the proposed framework captures principally new information. 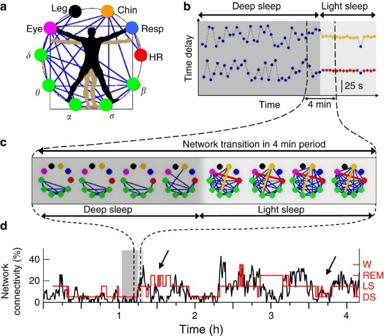Figure 1: Transitions in the network of physiological interactions. (a) Dynamical network of interactions between physiological systems where ten network nodes represent six physiological systems—brain activity (EEG waves:δ,θ,α,σandβ), cardiac (HR), respiratory (Resp), chin muscle tone, leg and eye movements. (b) Transition in the interactions between physiological systems across sleep stages. The time delay between two pairs of signals, (top)α-brain waves and chin muscle tone, and (bottom) HR and eye movement, quantifies their physiological interaction: highly irregular behaviour (blue dots) during deep sleep is followed by a period of TDS during light sleep indicating a stable physiological interaction (red dots for the HR–eye and orange dots for the α–chin interaction). (c) Transitions between physiological states are associated with changes in network topology: snapshots over 30-s windows during a transition from deep sleep (dark grey) to light sleep (light grey). During deep sleep, the network consists mainly of brain–brain links. With transition to light sleep, links between other physiological systems (network nodes) emerge and the network becomes highly connected. The stable α–chin and HR–eye interactions during light sleep in (b) are shown by an orange and a red network link, respectively. (d) Physiological network connectivity for one subject during night sleep calculated in 30-s windows as the fraction (%) of present links out of all possible links (brain–brain links not included, seeFig. 3e). Red line marks sleep stages as scored in a sleep lab. Low connectivity is consistently observed during deep sleep (0:30–1:15 h and 1:50–2:20 h) and REM sleep (1:30–1:45 h and 2:50–3:10 h), while transitions to light sleep and wake are associated with a significant increase in connectivity. Figure 1: Transitions in the network of physiological interactions. ( a ) Dynamical network of interactions between physiological systems where ten network nodes represent six physiological systems—brain activity (EEG waves: δ , θ , α , σ and β ), cardiac (HR), respiratory (Resp), chin muscle tone, leg and eye movements. ( b ) Transition in the interactions between physiological systems across sleep stages. The time delay between two pairs of signals, (top) α -brain waves and chin muscle tone, and (bottom) HR and eye movement, quantifies their physiological interaction: highly irregular behaviour (blue dots) during deep sleep is followed by a period of TDS during light sleep indicating a stable physiological interaction (red dots for the HR–eye and orange dots for the α–chin interaction). ( c ) Transitions between physiological states are associated with changes in network topology: snapshots over 30-s windows during a transition from deep sleep (dark grey) to light sleep (light grey). During deep sleep, the network consists mainly of brain–brain links. With transition to light sleep, links between other physiological systems (network nodes) emerge and the network becomes highly connected. The stable α–chin and HR–eye interactions during light sleep in ( b ) are shown by an orange and a red network link, respectively. ( d ) Physiological network connectivity for one subject during night sleep calculated in 30-s windows as the fraction (%) of present links out of all possible links (brain–brain links not included, see Fig. 3e ). Red line marks sleep stages as scored in a sleep lab. Low connectivity is consistently observed during deep sleep (0:30–1:15 h and 1:50–2:20 h) and REM sleep (1:30–1:45 h and 2:50–3:10 h), while transitions to light sleep and wake are associated with a significant increase in connectivity. 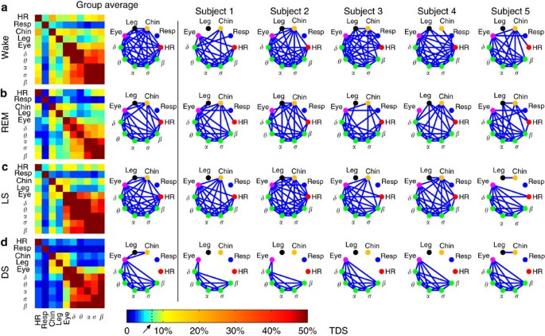Figure 2: Network connectivity across sleep stages. Group-averaged time delay stability (TDS) matrices and related networks of physiological interactions during different sleep stages: (a) wake; (b) REM sleep; (c) light sleep (LS); (d) deep sleep (DS). Matrix elements are obtained by quantifying the TDS for each pair of physiological systems after obtaining the weighted average of all subjects in the group:whereLiindicates the total duration of a given sleep stage for subjecti, andsiis the total duration of TDS withinLifor the considered pair of physiological signals. Colour code represents the average strength of interaction between systems quantified as the fraction of time (out of the total duration of a given sleep stage throughout the night) when TDS is observed. A network link between two systems is defined when their interaction is characterized by a TDS of⩾7% (arrow), a threshold determined by surrogate analysis (seeMethods). The physiological network exhibits transitions across sleep stages—lowest number of links during deep sleep (d), higher during REM (b), and highest during light sleep (c) and quiet wake (a)—a behaviour observed in the group-averaged network as well as for each subject. Network topology also changes with sleep-stage transitions: from predominantly brain–brain links during deep sleep to a high number of brain–periphery and periphery–periphery links during light sleep and wake. Full size image Figure 2: Network connectivity across sleep stages. Group-averaged time delay stability (TDS) matrices and related networks of physiological interactions during different sleep stages: ( a ) wake; ( b ) REM sleep; ( c ) light sleep (LS); ( d ) deep sleep (DS). Matrix elements are obtained by quantifying the TDS for each pair of physiological systems after obtaining the weighted average of all subjects in the group: where L i indicates the total duration of a given sleep stage for subject i , and s i is the total duration of TDS within L i for the considered pair of physiological signals. Colour code represents the average strength of interaction between systems quantified as the fraction of time (out of the total duration of a given sleep stage throughout the night) when TDS is observed. A network link between two systems is defined when their interaction is characterized by a TDS of ⩾ 7% (arrow), a threshold determined by surrogate analysis (see Methods ). The physiological network exhibits transitions across sleep stages—lowest number of links during deep sleep ( d ), higher during REM ( b ), and highest during light sleep ( c ) and quiet wake ( a )—a behaviour observed in the group-averaged network as well as for each subject. Network topology also changes with sleep-stage transitions: from predominantly brain–brain links during deep sleep to a high number of brain–periphery and periphery–periphery links during light sleep and wake. 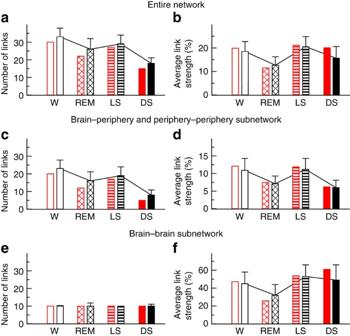Figure 3: Sleep-stage stratification pattern in network connectivity and network link strength. Group-averaged number of links (a) and averaged link strength (b) are significantly higher during wake and light sleep compared with REM and deep sleep (Studentt-testP<10−3for both quantities when comparing REM and deep sleep with wake and light sleep). There is no significant difference between wake and light sleep (P>5×10−2). This pattern is even more pronounced for the subnetwork formed by the brain–periphery and periphery–periphery links shown in (c) and (d) (P<10−6for both quantities when comparing REM and deep sleep with wake and light sleep). In contrast, the number of brain–brain links remains practically unchanged with sleep-stage transitions (e), and the average brain–brain link is ≈5 times stronger in all sleep stages compared with the other network links (f). The group-averaged patterns in the number of network links and in the average link strength across sleep stages (black bars) are consistent with the behaviour observed for individual subjects (red bars in all panels represent the same subject). The group-averaged number of links for each sleep stage is obtained from the corresponding group-averaged network inFig. 2. The average link strength is measured in % TDS and is obtained by taking the mean of all elements in the TDS matrix for each sleep stage (Fig. 2); it represents the average strength of all links in a network obtained from a given subject during a specific sleep stage, which then is averaged over all subjects. Error bars indicate s.d. obtained from a group of 36 subjects (Methods). Full size image Figure 3: Sleep-stage stratification pattern in network connectivity and network link strength. Group-averaged number of links ( a ) and averaged link strength ( b ) are significantly higher during wake and light sleep compared with REM and deep sleep (Student t -test P <10 −3 for both quantities when comparing REM and deep sleep with wake and light sleep). There is no significant difference between wake and light sleep ( P >5×10 −2 ). This pattern is even more pronounced for the subnetwork formed by the brain–periphery and periphery–periphery links shown in ( c ) and ( d ) ( P <10 −6 for both quantities when comparing REM and deep sleep with wake and light sleep). In contrast, the number of brain–brain links remains practically unchanged with sleep-stage transitions ( e ), and the average brain–brain link is ≈5 times stronger in all sleep stages compared with the other network links ( f ). The group-averaged patterns in the number of network links and in the average link strength across sleep stages (black bars) are consistent with the behaviour observed for individual subjects (red bars in all panels represent the same subject). The group-averaged number of links for each sleep stage is obtained from the corresponding group-averaged network in Fig. 2 . The average link strength is measured in % TDS and is obtained by taking the mean of all elements in the TDS matrix for each sleep stage ( Fig. 2 ); it represents the average strength of all links in a network obtained from a given subject during a specific sleep stage, which then is averaged over all subjects. Error bars indicate s.d. obtained from a group of 36 subjects (Methods). 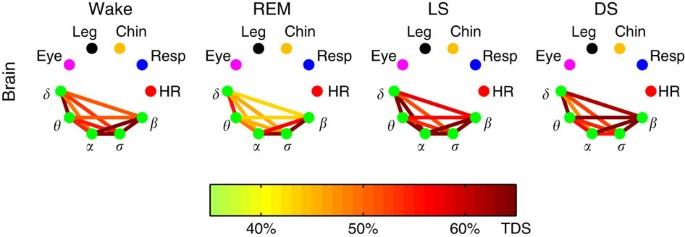Figure 4: Network connectivity and link strength of the brain–brain subnetwork for different sleep stages. While the topology of the brain subnetwork does not change, the strength of network links significantly changes with strongest links during light sleep and deep sleep (brown and dark red colour), intermediate during wake (red and orange colour) and weakest links during REM sleep (yellow colour). Full size image Figure 4: Network connectivity and link strength of the brain–brain subnetwork for different sleep stages. While the topology of the brain subnetwork does not change, the strength of network links significantly changes with strongest links during light sleep and deep sleep (brown and dark red colour), intermediate during wake (red and orange colour) and weakest links during REM sleep (yellow colour). 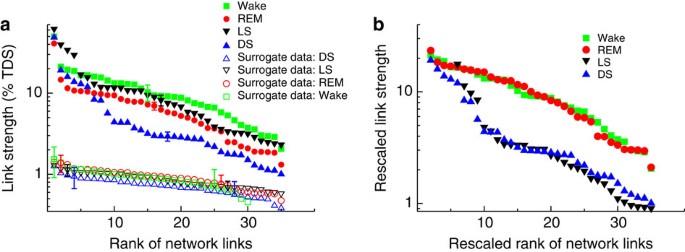Figure 5: Rank distributions of the strength of network links. Group-averaged strength of individual physiological network links for different sleep stages. Rank 1 corresponds to the strongest link in the network, that is, highest degree of time delay stability (TDS) (shown are all periphery–periphery and brain–periphery links). (a) The rank distributions for different sleep stages are characterized by different strength of the network links measured in % TDS—consistently lower values for most links during deep sleep, higher values during REM and highest during light sleep and wake, indicating that the stratification pattern inFig. 3dis present not only for the average link strength (when averaging over different types of links in the network) but also for the strength of individual links. Indeed, links from all ranks are consistently stronger in light sleep compared with deep sleep and REM: such rank-by-rank comparison of links across sleep stages is possible because the rank order of the links does not change significantly from one sleep stage to another (Wilcoxon signed-rank test for all pairs of rank distributions yields 0.77⩽P⩽0.93). A surrogate test based on TDS analysis of signals paired from different subjects, which eliminates endogenous physiological coupling, leads to significantly reduced link strength (P<10−3) and close to uniform rank distributions with no difference between sleep stages (open symbols), indicating that the TDS method uncovers physiologically relevant information. Error bars for the original and surrogate data indicate the standard error for a specific link when averaged over all 36 subjects or over 36 surrogate pairs respectively. (b) Rescaling the plots reveals two distinct forms of rank distributions: a slow decaying distribution for wake and REM, and a fast decaying distribution for light sleep and deep sleep with a pronounced plateau in the middle rank range corresponding to a cluster of links with similar strength, most of which are related to the cardiac system. Full size image Figure 5: Rank distributions of the strength of network links. Group-averaged strength of individual physiological network links for different sleep stages. Rank 1 corresponds to the strongest link in the network, that is, highest degree of time delay stability (TDS) (shown are all periphery–periphery and brain–periphery links). ( a ) The rank distributions for different sleep stages are characterized by different strength of the network links measured in % TDS—consistently lower values for most links during deep sleep, higher values during REM and highest during light sleep and wake, indicating that the stratification pattern in Fig. 3d is present not only for the average link strength (when averaging over different types of links in the network) but also for the strength of individual links. Indeed, links from all ranks are consistently stronger in light sleep compared with deep sleep and REM: such rank-by-rank comparison of links across sleep stages is possible because the rank order of the links does not change significantly from one sleep stage to another (Wilcoxon signed-rank test for all pairs of rank distributions yields 0.77 ⩽ P ⩽ 0.93). A surrogate test based on TDS analysis of signals paired from different subjects, which eliminates endogenous physiological coupling, leads to significantly reduced link strength ( P <10 −3 ) and close to uniform rank distributions with no difference between sleep stages (open symbols), indicating that the TDS method uncovers physiologically relevant information. Error bars for the original and surrogate data indicate the standard error for a specific link when averaged over all 36 subjects or over 36 surrogate pairs respectively. ( b ) Rescaling the plots reveals two distinct forms of rank distributions: a slow decaying distribution for wake and REM, and a fast decaying distribution for light sleep and deep sleep with a pronounced plateau in the middle rank range corresponding to a cluster of links with similar strength, most of which are related to the cardiac system. 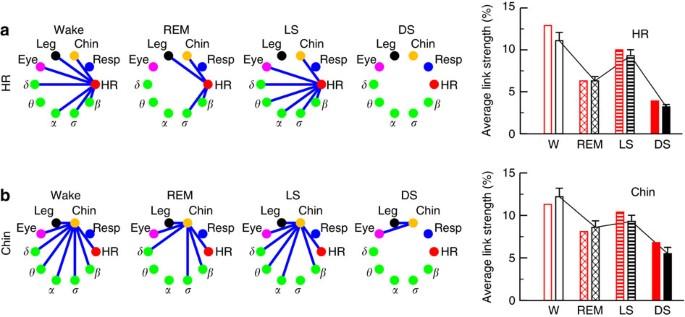Figure 6: Transitions in connectivity and link strength of individual network nodes across sleep stages. The number of links to specific network nodes significantly changes, with practically no links during deep sleep, a few links during REM and much higher connectivity during light sleep and wake. Notably, the average strength of the links connecting a given network node is also lowest during deep sleep and highest during light sleep and wake. Shown are connectivity and average link strength for two network nodes: (a) heart and (b) chin. This sleep-stage stratification pattern in individual node connectivity and in the average strength of the links connecting a specific network node is consistent with the transitions of the entire network across sleep stages shown inFig. 3 c,d. Networks for (a) heart and (b) chin are obtained by averaging the corresponding networks for all subjects. During deep sleep, no links to the heart are shown as the strength of each link averaged over all subjects is below the significance threshold (Figs 2and7, Methods). Right bars in the panels represent for different sleep stages the group mean of the average strength of network links connecting the heart and chin, respectively, and error bars show the s.d. obtained from a group of 36 subjects (Methods). Left bars represent an individual subject. Note that the absence of a link between heart rate and respiration in the physiological network does not indicate absence of cardio–respiratory coupling but rather that this coupling as represented by time delay stability (TDS) is rarely stable for periods longer than 2–4 min (where 2 min is the minimum window over which TDS is determined; Method section), and that cardio–respiratory TDS episodes form <7% of the recordings, which is the significance threshold level (Method section). Such 'on' and 'off' intermittent interaction between these two systems is observed also in other independent measures of cardio–respiratory coupling—respiratory sinus arrhythmia (RSA)41,42and the degree of phase synchronization6—where relatively short 'on' episodes are separated by periods of no interrelation as quantified by these measures. Full size image Figure 6: Transitions in connectivity and link strength of individual network nodes across sleep stages. The number of links to specific network nodes significantly changes, with practically no links during deep sleep, a few links during REM and much higher connectivity during light sleep and wake. Notably, the average strength of the links connecting a given network node is also lowest during deep sleep and highest during light sleep and wake. Shown are connectivity and average link strength for two network nodes: ( a ) heart and ( b ) chin. This sleep-stage stratification pattern in individual node connectivity and in the average strength of the links connecting a specific network node is consistent with the transitions of the entire network across sleep stages shown in Fig. 3 c,d . Networks for ( a ) heart and ( b ) chin are obtained by averaging the corresponding networks for all subjects. During deep sleep, no links to the heart are shown as the strength of each link averaged over all subjects is below the significance threshold ( Figs 2 and 7 , Methods). Right bars in the panels represent for different sleep stages the group mean of the average strength of network links connecting the heart and chin, respectively, and error bars show the s.d. obtained from a group of 36 subjects (Methods). Left bars represent an individual subject. Note that the absence of a link between heart rate and respiration in the physiological network does not indicate absence of cardio–respiratory coupling but rather that this coupling as represented by time delay stability (TDS) is rarely stable for periods longer than 2–4 min (where 2 min is the minimum window over which TDS is determined; Method section), and that cardio–respiratory TDS episodes form <7% of the recordings, which is the significance threshold level (Method section). Such 'on' and 'off' intermittent interaction between these two systems is observed also in other independent measures of cardio–respiratory coupling—respiratory sinus arrhythmia (RSA) [41] , [42] and the degree of phase synchronization [6] —where relatively short 'on' episodes are separated by periods of no interrelation as quantified by these measures. Full size image To quantify the interaction between physiological systems and to probe how this interaction changes in time under different physiological conditions, we study the time delay with which modulations in the output dynamics of a given physiological system are consistently followed by corresponding modulations in the signal output of another system. Periods of time with approximately constant time delay indicate a stable physiological interaction, and stronger coupling between physiological systems results in longer periods of TDS. Utilizing the TDS method, we build a dynamical network of physiological interactions, where network links between physiological systems (considered as network nodes) are established when the TDS representing the coupling of these systems exceeds a significance threshold level, and where the strength of the links is proportional to the percentage of time for which TDS is observed (Methods). Transitions in network topology with physiological function We apply this new approach to a group of healthy young subjects (Methods). We find that the network of interactions between physiological systems is very sensitive to sleep-stage transitions. In a short time window of just a few minutes, the network topology can dramatically change—from only a few links to a multitude of links ( Fig. 1 )—indicating transitions in the global interconnectivity between physiological systems. These network transitions are not associated with random occurrence or loss of links but are characterized by certain organization in network topology where given links between physiological systems remain stable during the transition while others do not—for example, brain–brain links persist during the transition from deep sleep to light sleep while brain–periphery links significantly change ( Fig. 1c ). Further, we find that sleep-stage transitions are paralleled by abrupt jumps in the total number of links leading to higher or lower network connectivity ( Fig. 1c,d ). These network dynamics are observed for each subject in the database, where consecutive episodes of sleep stages are paralleled by a level of connectivity specific for each sleep stage, and where sleep-stage transitions are consistently followed by transitions in network connectivity throughout the course of the night ( Fig. 1d ). Indeed, the network of physiological interactions exhibits a remarkable responsiveness as network connectivity changes even for short sleep-stage episodes (arrows in Fig. 1d ), demonstrating a robust relationship between network topology and function. This is the first observation of a real network evolving in time and undergoing topological transitions from one state to another. To identify the characteristic network topology for each sleep stage, we obtain group-averaged TDS matrices, where each matrix element represents the percentage of time with stable time delay between two physiological systems, estimated over all episodes of a given sleep stage throughout the night. Matrix elements above a threshold of statistical significance ( Fig. 7 , Methods) indicate stable interactions between physiological systems represented by network links ( Fig. 2 ). We find that matrix elements greatly vary for different sleep stages with much higher values for wake and light sleep, lower values for REM and lowest for deep sleep. This is reflected in higher network connectivity for wake and light sleep, lower for REM and significantly reduced number of links during deep sleep ( Fig. 3a ). Further, the TDS matrices indicate separate subgroups of interactions between physiological systems—brain–periphery, periphery–periphery and brain–brain interactions—that are affected differently during sleep stages and form different subnetworks. Specifically, matrix elements representing interactions between peripheral systems (cardiac, respiratory, chin, eye and leg) and the brain as well as interactions among the peripheral systems are very sensitive to sleep-stage transitions, leading to different network topology for different sleep stages ( Fig. 2 ). We find subnetworks with high number of brain–periphery and periphery–periphery links during wake and light sleep, lower number of links during REM and a significant reduction of links at deep sleep ( Fig. 3c ). In contrast, matrix elements representing brain–brain interactions form a subnetwork with the same number of brain–brain links ( Fig. 3e ), and stable topology is consistently present in the physiological network during all sleep stages ( Fig. 2 ). Sleep-stage-related transitions in network connectivity and topology are not only present in the group-averaged data but also in the physiological networks of individual subjects, suggesting universal behaviour ( Fig. 2 ). Notably, we find a higher number of brain–periphery links during REM compared with deep sleep despite the inhibition of motoneurons in the brain leading to muscle atonia during REM [29] . The empirical observations of significant difference in network connectivity and topology during light sleep compared with deep sleep are surprising, given the similarity in spectral, scale-invariant and nonlinear properties of physiological dynamics during light sleep and deep sleep [3] , [4] , [25] , [26] (both stages traditionally classified as non-rapid eye movement sleep (NREM)), and indicate that previously unrecognized aspects of sleep regulation may be involved in the control of physiological network interactions. 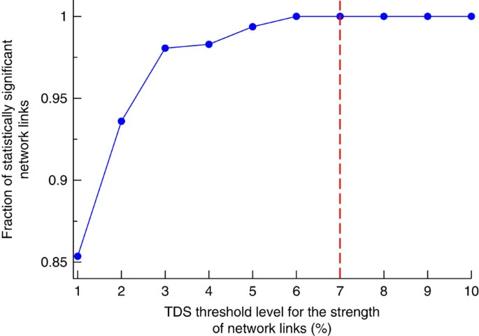Figure 7: Determining significance threshold for the strength of network links. With increasing the time delay stability (TDS) threshold level that allows only stronger links with higher TDS values to be considered in the physiological network, the fraction of statistically significant network links that carry physiologically relevant information also increases, and at a significance threshold of ≈7% TDS (marked by a vertical dashed line) all network links (100%) are statistically significant. Periphery–periphery and brain–periphery links during all sleep stages are considered when determining this threshold. Statistical significance of a specific physiological link is estimated by comparing the strength distribution of this link across all subjects in the group with a distribution of surrogate links representing 'interactions' between the same systems paired from different subjects. Based on this surrogate test, aP-value <10−3obtained from the Studentt-test indicates statistically significant strength of a given link. Figure 7: Determining significance threshold for the strength of network links. With increasing the time delay stability (TDS) threshold level that allows only stronger links with higher TDS values to be considered in the physiological network, the fraction of statistically significant network links that carry physiologically relevant information also increases, and at a significance threshold of ≈7% TDS (marked by a vertical dashed line) all network links (100%) are statistically significant. Periphery–periphery and brain–periphery links during all sleep stages are considered when determining this threshold. Statistical significance of a specific physiological link is estimated by comparing the strength distribution of this link across all subjects in the group with a distribution of surrogate links representing 'interactions' between the same systems paired from different subjects. Based on this surrogate test, a P -value <10 −3 obtained from the Student t -test indicates statistically significant strength of a given link. Full size image Physiological states and network link strength stratification Networks with identical connectivity and topology can exhibit different strength of their links. Network link strength is determined as the fraction of time when TDS is observed (Methods). We find that the average strength of network links changes with sleep-stage transitions: network links are significantly stronger during wake and light sleep compared with REM and deep sleep—a pattern similar to the behaviour of the network connectivity across sleep stages ( Fig. 3a,b ). Further, subnetworks of physiological interactions exhibit different relationship between connectivity and average link strength. Specifically, the subnetwork of brain–periphery and periphery–periphery interactions is characterized by significantly stronger links (and also higher connectivity) during wake and light sleep, and much weaker links (with lower network connectivity) during deep sleep and REM ( Fig. 3c,d ). In contrast, the subnetwork of brain–brain interactions exhibits very different patterns for the connectivity and the average link strength—while the group average subnetwork connectivity remains constant across sleep stages, the average link strength varies with highest values during light sleep and deep sleep, and a dramatic ≈40% decline during REM. The observation of significantly stronger links in the brain–brain subnetwork during NREM compared with REM sleep is consistent with the characteristic of NREM as EEG-synchronized sleep and REM as EEG-desynchronized sleep [29] . During NREM sleep, adjacent cortical neurons fire synchronously with a relatively low-frequency rhythm [30] leading to coherence between frequency bands in the EEG signal, and thus to stable time delays and strong network links ( Fig. 3f ). In contrast, during REM sleep cortical neurons are highly active but fire asynchronously [30] , resulting in weaker links ( Fig. 3f ). Our findings of stronger links in the brain–brain subnetwork during non-REM sleep ( Figs 3f and 4 ) indicate that bursts (periods of sudden temporal increase) in the spectral power of one EEG-frequency band are consistently synchronized in time with bursts in a different EEG-frequency band, thus leading to longer periods of TDS and correspondingly stronger network links. This can explain some seemingly surprising network links—for example, we find a strong link between α and δ brain activity during non-REM sleep ( Fig. 2 ) although α waves are greatly diminished and δ waves are dominant [29] . As the spectral densities of both waves are normalized before the TDS analysis (Methods), the presence of a stable α – δ link indicates that a relative increase in the spectral density in one wave is followed, with a stable time delay, by a corresponding increase in the density of the other wave—an intriguing physiological interaction that persists not only during deep sleep but is also present in light sleep, REM and quiet wake ( Fig. 2 ). Notably, the average link strength of the brain–brain subnetwork is by a factor of ≈5 higher compared with all other links in the physiological network ( Fig. 3d,f ). The finding of completely different sleep-stage stratification patterns in key network properties of the brain–brain subnetwork compared with the periphery–periphery/brain–periphery subnetworks suggests a very different role these subnetworks have in coordinating physiological interactions during sleep. The similarity in the brain–brain subnetwork during deep sleep and light sleep indicates that the proposed TDS approach is sensitive to quantify synchronous slow-wave brain activity during NREM sleep that leads to stronger brain–brain links during light sleep and deep sleep (≈50–60% TDS) compared with REM (≈35% TDS), as shown in Figs 3f and 4 . The significant difference between light sleep and deep sleep observed for the periphery–periphery/brain–periphery subnetwork in the number of links ( t -test: P <10 −12 ) as well as in the average link strength ( t -test: P <10 −11 ) indicates that the interactions between physiological dynamics outside the brain are very different during these sleep stages. Our finding that the average link strength exhibits a specific stratification pattern across sleep stages ( Fig. 3 ) raises the question whether the underlying distribution of the network links strength is also sleep-stage dependent. To this end we probe the relative strength of individual links, and we obtain the rank distribution of the strength of network links for each sleep stage averaged over all subjects in the group ( Fig. 5a ). We find that the rank distribution corresponding to deep sleep is vertically shifted to much lower values for the strength of the network links, while the rank distribution for light sleep and wake is for all links consistently higher than the distribution for REM. Thus, the sleep-stage stratification pattern we find for the average strength of the network links ( Fig. 3d ) originates from the systematic change in the strength of individual network links with sleep-stage transitions. Notably, while the strength of individual network links changes significantly with sleep stages, the rank order of the links does not significantly change. After rescaling the rank distributions for light sleep and REM (by horizontal and vertical shifts), we find that they collapse onto the rank plots of deep sleep and wake, respectively, following two distinct functional forms: a slow and smoothly decaying rank distribution for REM and wake, and a much faster decaying rank distribution for deep sleep and light sleep with a characteristic plateau in the mid rank range indicating a cluster of links with similar strength ( Fig. 5b ). We note that, although the form of the rank distributions for deep sleep and light sleep as well as for wake and REM are, respectively, very similar, the average strength of the links is significantly different between deep sleep and light sleep and between wake and REM ( Fig. 3d ). Local topology and connectivity of the physiological network Our observations that physiological networks undergo dynamic transitions where key global properties significantly change with sleep-stage transitions raise the question whether local topology and connectivity of individual network nodes also change during these transitions. Considering each physiological system (network node) separately, we examine the number and strength of all links connecting the system with the rest of the network. Specifically, we find that the cardiac system is highly connected to other physiological systems in the network during wake and light sleep ( Fig. 6 ). In contrast, during deep sleep we do not find statistically significant TDS in the interactions of the cardiac system, which is reflected by absence of cardiac links ( Fig. 6 ). Further, we find that the average strength of the links connected to the cardiac system also changes with sleep stages: stronger interactions (high % TDS) during wake and light sleep, and significantly weaker interactions below the significance threshold during deep sleep ( Fig. 6 ). Such 'isolation' of the cardiac node from the rest of the network indicates a more autonomous cardiac function during deep sleep—also supported by earlier observations of breakdown of long-range correlations and close to random behaviour in heartbeat intervals in this sleep stage [3] . Transition to light sleep, REM and wake, where the average link strength and connectivity of the cardiac system is significantly higher indicating increased interactions with the rest of the network, leads to correspondingly higher degree of correlations in cardiac dynamics [3] . Similarly, respiratory dynamics also exhibit high degree of correlations during REM and wake, lower during light sleep and close to random behaviour during deep sleep [26] . We also find such transitions in the number and strength of links across sleep stages for other network nodes ( Fig. 6 ). Moreover, the sleep-stage stratification pattern in connectivity and average link strength for individual network nodes ( Fig. 6 ) is consistent with the pattern we observe for the entire network ( Fig. 3 ). Our findings of significant reduction in the number and strength of brain–periphery and periphery–periphery links in the corresponding subnetworks during deep sleep indicate that breakdown of cortical interactions, previously reported during deep sleep [31] , may also extend to other physiological systems under neural regulation. Indeed, the low connectivity in the physiological network we find in deep sleep may explain why people awakened during deep sleep do not adjust immediately and often feel groggy and disoriented for a few minutes. This effect is not observed if subjects are awakened from light sleep [29] when we find the physiological network to be highly connected ( Fig. 2 ). Further, as risk of predation modifies sleep architecture [32] , [33] , [34] and as abrupt awakening from deep sleep is associated with increased sleep inertia, higher sensory threshold, and impaired sensory reaction and performance [35] , [36] that may lead to increased vulnerability, the fact that deep sleep (lowest physiological network connectivity) dominates at the beginning of the night and not close to dawn, when many large predators preferably hunt, may have been evolutionarily advantageous. Introducing a framework based on the concept of TDS, we identify a robust network of interactions between physiological systems, which remains stable across subjects during a given physiological state. Further, changes in the physiological state lead to complex network transitions associated with a remarkably structured reorganization of network connectivity and topology that simultaneously occurs in the entire network as well as at the level of individual network nodes, while preserving the hierarchical order in the strength of individual network links. Such network transitions lead to the formation of subnetworks of physiological interactions with different topology and dynamical characteristics. In the context of sleep stages, network transitions are characterized by a specific stratification pattern where network connectivity and link strength are significantly higher during light sleep compared with deep sleep and during wake compared with REM. This cannot be explained by the dynamical characteristics of the output signals from individual physiological systems, which are similar during light sleep and deep sleep as well as during wake and REM. The dramatic change in network structure with transition from one physiological state to another within a short time window indicates a high flexibility in the interaction between physiological systems in response to change in physiological regulation. Such change in network structure in response to change in the mechanisms of control during different physiological states suggests that our findings reflect intrinsic features of physiological interaction. The observed stability in network topology and rank order of links strength during sleep stages, and the transitions in network organization across sleep stages provide new insight into the role that individual physiological systems as well as their interactions have during specific physiological states. While our study is limited to a data-driven approach, these empirical findings may facilitate future efforts on developing and testing network models of physiological interaction. This system-wide integrative approach to individual systems and the network of their interactions may facilitate the emergence of a new dimension to the field of systems physiology [7] that will include not only interactions within but also across physiological systems. In relation to critical clinical care, where multiple organ failure is often the reason for fatal outcome [24] , [37] , our framework may have practical utility in assessing whether dynamical links between physiological systems remain substantially altered even when the function of specific systems is restored after treatment [38] . While we demonstrate one specific application, the framework we develop can be applied to a broad range of complex systems where the TDS method can serve as a tool to characterize and understand the dynamics and function of real-world heterogeneous and interdependent networks. The established relationship between dynamical network topology and network function has not only significant medical and clinical implications, but is also of relevance for the general theory of complex networks. Data We analyse continuously recorded multichannel physiological data obtained from 36 healthy young subjects (18 female, 18 male, with ages between 20–40, average 29 years) during night-time sleep [39] (average record duration is 7.8 h). This allows us to track the dynamics and evolution of the network of physiological interactions during different sleep stages and sleep-stage transitions ( Fig. 1 ). We focus on physiological dynamics during sleep as sleep stages are well-defined physiological states, and external influences due to physical activity or sensory inputs are reduced during sleep. Sleep stages are scored in 30s epochs by sleep lab technicians based on standard criteria. In particular, we focus on the EEG, the electrocardiogram, respiration, the electrooculogram, and the electromyogram of the chin and leg. In order to compare these very different signals with each other and to study interrelations between them, we extract the following time series from the raw signals: the spectral power of five frequency bands of the EEG in moving windows of 2 s with a 1 s overlap: δ waves (0.5–3.5 Hz), θ waves (4–7.5 Hz), α waves (8–11.5 Hz), σ waves (12–15.5 Hz) and β waves (16–19.5 Hz); the variance of the electrooculogram and electromyogram signals in moving windows of 2 s with a 1s overlap; heartbeat RR intervals and interbreath intervals are both re-sampled to 1 Hz (1 s bins) after which values are inverted to obtain heart rate and respiratory rate. Thus, all time series have the same time resolution of 1 s before the TDS analysis is applied. Utilizing sleep data as an example, we demonstrate that a network approach to physiological interactions is necessary to understand how modulations in the regulatory mechanism of individual systems translate into reorganization of physiological interactions across the human organism. TDS method Integrated physiological systems are coupled by feedback and/or feedforward loops with a broad range of time delays. To probe physiological coupling, we propose an approach based on the concept of TDS: in the presence of stable/strong interactions between two systems, transient modulations in the output signal of one system lead to corresponding changes that occur with a stable time lag in the output signal of another coupled system. Thus, long periods of constant time delay indicate strong physiological coupling. The TDS method we developed for this study consists of the following steps: To probe the interaction between two physiological systems X and Y, we consider their output signals { x } and { y } each of length N . We divide both signals { x } and { y } into N L -overlapping segments v of equal length L =60 s. We choose an overlap of L /2=30 s, which corresponds to the time resolution of the conventional sleep-stage-scoring epochs, and thus N L =[2 N/L ]−1. Before the analysis, the signal in each segment v is normalized separately to zero mean and unit standard deviation, in order to remove constant trends in the data and to obtain dimensionless signals. This normalization procedure assures that the estimated coupling between the signals { x } and { y } is not affected by their relative amplitudes. Next, we calculate which is the cross-correlation function within each segment v =1,..., N L by applying periodic boundary conditions. For each segment v , we define the time delay τ 0 v to correspond to the maximum in the absolute value of the cross-correlation function C v xy ( τ ) in this segment Time periods of stable interrelation between two signals are represented by segments of approximately constant τ 0 (light shade region in Fig. 1b ) in the newly defined series of time delays, In contrast, absence of stable coupling between the signals corresponds to large fluctuations in τ 0 (dark shade region in Fig. 1b ). We identify two systems as linked if their corresponding signals exhibit a time delay that does not change by more than ±1 s for several consecutive segments v . We track the values of τ 0 along the series { τ 0 v }: when for at least four out of five consecutive segments v (corresponding to a window of 5×30 s) the time delay remains in the interval [ τ 0 −1, τ 0 +1], these segments are labelled as stable. This procedure is repeated for a sliding window with a step size one along the entire series { τ 0 v }. The % TDS is finally calculated as the fraction of stable points in the time series { τ 0 v }. Longer periods of TDS between the output signals of two systems reflect more stable interaction/coupling between these systems. Thus, the strength of the links in the physiological network is determined by the percentage of time when TDS is observed: higher percentage of TDS corresponds to stronger links. To identify physiologically relevant interactions, represented as links in the physiological network, we determine a significance threshold level for the TDS based on comparison with surrogate data: only interactions characterized by TDS values above the significance threshold are considered. The TDS method is general, and can be applied to diverse systems. It is more reliable in identifying physiological coupling compared with traditional cross-correlation and cross-coherence analyses ( Fig. 8 ), which are not suitable for heterogeneous and non-stationary signals, and are affected by the degree of auto-correlations in these signals [40] . 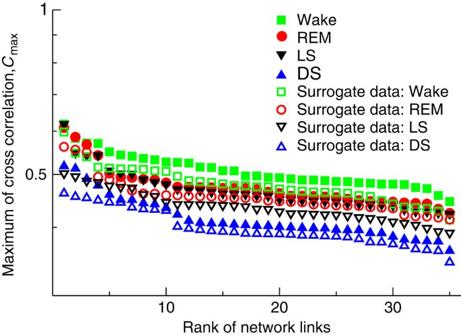Figure 8: Cross-correlation and surrogate analysis. Rank plots obtained from cross-correlation analysis show no statistically significant differences between real and surrogate data, indicating that cross-correlation is not a reliable measure to identify physiological interactions. Figure 8: Cross-correlation and surrogate analysis. Rank plots obtained from cross-correlation analysis show no statistically significant differences between real and surrogate data, indicating that cross-correlation is not a reliable measure to identify physiological interactions. Full size image To compare interactions between physiological systems that are very different in strength and vary with change of physiological state (for example, transitions across sleep stages), we define the significance threshold as the percentage of TDS for which all links included in the physiological network are statistically significant. To identify statistical significance of a given link between two physiological systems, we compare the distribution of TDS values for this link obtained from all 36 subjects in our database with the distribution of TDS values obtained for 100 surrogates of this link where the signal outputs from the same two physiological systems taken from different subjects are paired for the analysis in order to eliminate the endogenous physiological coupling. A Student t -test was performed to determine the statistical significance between the two distributions. This procedure is repeated for all pairs of systems (links) in the network, and network links are identified as significant when the t -test P -value <10 −3 . The significance threshold level for TDS is then defined as the value above which all network links are statistically significant, and thus represent endogenous interactions between physiological systems. We find that a threshold of ∼ 7% TDS is needed to identify networks of statistically significant links for all sleep stages ( Fig. 7 ). Surrogate tests To confirm that the TDS method captures physiologically relevant information about the endogenous interactions between systems, we perform a surrogate test where we pair physiological signals from different subjects, thus eliminating physiological coupling. Applying the TDS method to these surrogate data, we obtain almost uniform rank distributions with significantly decreased link strength ( Fig. 5a ) due to the absence of physiological interactions. Further, all surrogate distributions conform to a single curve, indicating that the sleep-stage stratification we observe for the real data reflects indeed changes in physiological coupling with sleep-stage transitions. In contrast, the same surrogate test applied to traditional cross-correlation analysis does not show a difference between the rank distributions from surrogate and real data ( Fig. 8 ). We find that the TDS method is better suited than the traditional cross-correlation analysis in identifying networks of endogenous physiological interactions. Rank plots obtained from cross-correlation analysis ( Fig. 8 ) show that the cross-correlation strength C max (global maximum of the cross-correlation function) is consistently lower for all links during deep sleep, higher for light sleep and REM, and highest during wake—a stratification related to the gradual increase in the strength of autocorrelations in the signal output of physiological systems [3] , [26] , which in turn increases the degree of cross-correlations [40] . Surrogate tests based on pairs of signals from different subjects, where the coupling between systems is abolished but physiological autocorrelations are preserved, show no statistical difference between the surrogate (open symbols) and original (filled symbols) rank distributions of C max , suggesting that in this context cross-correlations do not provide physiologically relevant information regarding the interaction between systems. Indeed, even for uncoupled systems, high autocorrelations in the output signals lead to spurious detection of cross-correlations [40] . In contrast, the TDS method is not affected by the autocorrelations—surrogate rank plots for different sleep stages collapse and do not exhibit vertical stratification as shown in Fig. 5a . To test the robustness of the stratification pattern in network topology and connectivity across sleep stages (shown in Figs 2 and 3 ), we repeat our analyses for two additional thresholds: 5% TDS and 9% TDS. With increasing the threshold for TDS from 5 to 9%, the overall number of links in the network decreases (compare Fig. 9a,c,e with Fig. 9b,d,f ). However, the general sleep-stage stratification pattern is preserved with highest number of links during light sleep and wake, lower during REM, and significant reduction in network connectivity during deep sleep ( Fig. 9 ). The stability of the observed pattern in network connectivity for a relatively broad range around the significance threshold of 7% TDS indicates that the identified network is a robust measure of physiological interactions. 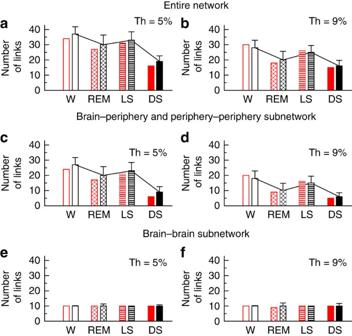Figure 9: Stability of sleep-stage stratification pattern in network connectivity. Group-averaged number of network links for two different thresholds (Th) during wake, REM, light and deep sleep. Results for threshold of Th=5% time delay stability (TDS) are shown ina,cande, and results for threshold of Th=9% TDS are shown inb,dandf. The sleep-stage stratification pattern observed for the significance threshold of 7% TDS (shown inFig. 3) is preserved also for thresholds of 5 and 9% TDS, indicating stability of the results. Note that the number of links in the brain–brain subnetwork remains unchanged for different sleep stages (e, f) as the strength of all links in this subnetwork is well above 9% TDS (Fig. 3f). Figure 9: Stability of sleep-stage stratification pattern in network connectivity. Group-averaged number of network links for two different thresholds (Th) during wake, REM, light and deep sleep. Results for threshold of Th=5% time delay stability (TDS) are shown in a , c and e , and results for threshold of Th=9% TDS are shown in b , d and f . The sleep-stage stratification pattern observed for the significance threshold of 7% TDS (shown in Fig. 3 ) is preserved also for thresholds of 5 and 9% TDS, indicating stability of the results. Note that the number of links in the brain–brain subnetwork remains unchanged for different sleep stages ( e, f ) as the strength of all links in this subnetwork is well above 9% TDS ( Fig. 3f ). Full size image How to cite this article: Bashan, A. et al . Network Physiology reveals relations between network topology and physiological function. Nat. Commun. 3:702 doi: 10.1038/ncomms1705 (2012).